A novel liquid organic hydrogen carrier system based on catalytic peptide formation and hydrogenation Hydrogen is an efficient green fuel, but its low energy density when stored under high pressure or cryogenically, and safety issues, presents significant disadvantages; hence finding efficient and safe hydrogen carriers is a major challenge. Of special interest are liquid organic hydrogen carriers (LOHCs), which can be readily loaded and unloaded with considerable amounts of hydrogen. However, disadvantages include high hydrogen pressure requirements, high reaction temperatures for both hydrogenation and dehydrogenation steps, which require different catalysts, and high LOHC cost. Here we present a readily reversible LOHC system based on catalytic peptide formation and hydrogenation, using an inexpensive, safe and abundant organic compound with high potential capacity to store and release hydrogen, applying the same catalyst for loading and unloading hydrogen under relatively mild conditions. Mechanistic insight of the catalytic reaction is provided. We believe that these findings may lead to the development of an inexpensive, safe and clean liquid hydrogen carrier system. Containing the highest energy density per unit mass and producing only water upon combustion, hydrogen is a most efficient and environmentally friendly fuel [1] , [2] , [3] , [4] . In fact, the concept of a ‘hydrogen economy’ was suggested as early as 1972 (ref. 5 ). However, the low energy density of hydrogen stored in high-pressure tanks or as a liquid in cryogenic tanks, and potential safety issues, presents significant disadvantages. Thus, finding suitable hydrogen carriers is highly desirable [1] , [2] , [3] , [4] , [6] , [7] . For decades, scientists have searched for suitable hydrogen storage materials, such as main-group hydrides, metal organic frameworks, metal clusters and nanostructured materials. Unfortunately, all these systems suffer from significant limitations [1] , [2] , [3] , [4] . Recently, organic compounds, such as formic acid [8] , methanol–water [9] , [10] , [11] , [12] , formaldehyde–water [13] , alcohols [14] and carbohydrates [15] , were intensively studied as potential hydrogen storage systems. Of special interest are ‘liquid organic hydrogen carriers’ (LOHCs), which can be readily dehydrogenated as well as regenerated, with considerable hydrogen capacity and that might be used for transportation and stationary purposes [7] , [16] , [17] , [18] , [19] , [20] . An attractive LOHC of potential commercial interest has been N -ethylcarbazole [16] , [17] , [18] , which upon hydrogenation to perhydro- N -ethylcarbazole consumes 6 equivalents (equiv.) of H 2 , resulting in a hydrogen storage capacity as high as 5.8 wt%. However, disadvantages of this system include the requirement of high H 2 pressure for the hydrogenation step, and high reaction temperature for both the hydrogenation and dehydrogenation steps, for which different catalysts are required [17] , [18] . Two other recent examples of LOHCs are 2-methyl-1,2,3,4-tetrahydroquinoline and 2,6-dimethyldecahydro-1,5-naphthyridine, which can be reversibly dehydrogenated to 2-methylquinoline and 2,6-dimethyl-1,5-naphthyridine, respectively, catalysed by Ir complexes. However, these systems suffer from very high catalyst loading (5 mol%), high cost of iridium, relatively expensive liquids and low hydrogen storage capacity of 2-methyl-1,2,3,4-tetrahydroquinoline [19] , [20] . Clearly, discovery of LOHC systems based on inexpensive and abundant organic compounds with high capacity to store and release hydrogen, ideally using the same catalyst for both loading and unloading hydrogen under relatively mild conditions, and compatible with existing infrastructure for transport and refuelling, is a major challenge. Here we report a promising LOHC system, based on the inexpensive, abundant 2-aminoethanol (AE), that is catalytically converted to a cyclic dipeptide with formation of hydrogen gas by use of a ruthenium pincer catalyst; peptide hydrogenation, using the same catalyst, regenerates AE. Mechanistic information regarding this conceptually new LOHC system is provided. Use of AE as LOHC We reported the PNN ruthenium pincer complexes 1 – 4 ( Fig. 1a ) that efficiently catalyse several C–O and C–N bond forming dehydrogenative coupling reactions, giving pure hydrogen as the sole byproduct [21] , [22] , [23] , [24] , [25] , and also the reverse hydrogenation reactions [22] , [26] . For example, the dearomatized catalyst 2 directly produces amides from alcohols and amines with the liberation of H 2 (ref. 24 ). Complex 2 can be obtained in situ by the deprotonation of complex 1 with a base. The reverse reaction, hydrogenation of amides to form alcohols and amines, was also achieved under mild hydrogen pressure using the same catalyst ( Fig. 1b ; ref. 26 ). These two reactions suggest the potential for loading and unloading H 2 using amines and alcohols. A particularly attractive compound is AE; as an amine and an alcohol, one molecule of AE will release two molecules of H 2 if piperazine-2,5-dione (glycine anhydride, GA) can be obtained ( Fig. 1c ), resulting in high potential hydrogen storage capacity of 6.56 wt%. In addition, since it is industrially produced in large amounts (for CO 2 scrubbing) [27] , AE is very inexpensive and readily available. 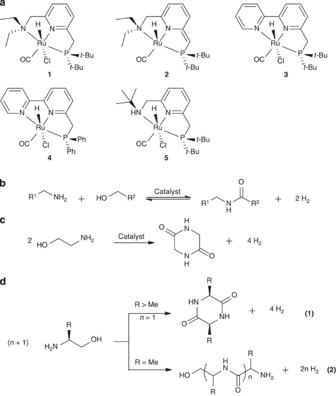Figure 1: Dehydrogenative amidation reactions catalysed by PNN ruthenium pincer complexes. (a) Complexes1–5, (b) reversible dehydrogenative cross-coupling of amines and alcohols to produce amides, (c) unknown dehydrogenation of AE to produce GA and H2, and (d) formation of cyclic dipeptides (1) and oligopeptides (2) fromβ-aminoalcohols. Figure 1: Dehydrogenative amidation reactions catalysed by PNN ruthenium pincer complexes. ( a ) Complexes 1 – 5 , ( b ) reversible dehydrogenative cross-coupling of amines and alcohols to produce amides, ( c ) unknown dehydrogenation of AE to produce GA and H 2 , and ( d ) formation of cyclic dipeptides (1) and oligopeptides (2) from β -aminoalcohols. Full size image Hydrogen generation experiments We recently reported that aminoalcohols can undergo dehydrogenative coupling to form cyclic dipeptides (diketopiperazines) and/or oligopeptides ( Fig. 1d ), depending on the substituent R [25] ; in case of R=Me (( S )-2-aminopropan-1-ol), linear oligopeptides are formed, while with larger substituents diketopiperazines are the major products. Density functional theory (DFT) calculations that we have performed show that conversion of AE to GA or to linear oligopeptides are both thermodynamically favourable processes, but the latter is thermodynamically more favoured. For the reaction in Fig. 1c , the calculated Gibbs free energy (Δ G 298 ) is −6.08 kcal mol −1 ; for reaction (2) in Fig. 1d (R=H), Δ G 298 is −10.17 kcal mol −1 ( n =3), −18.18 kcal mol −1 ( n =6) and −40.19 kcal mol −1 ( n =11; see Supplementary Fig. 1 , Supplementary Tables 1 and 2 , and Supplementary Discussion for full computational details). However, formation of linear oligopeptides as the major products is less beneficial since this lowers the hydrogen storage capacity of AE. On the other hand, the hydrogen storage capacity of linear peptides can also be considerable. For example, in Fig. 1d (R=H), reaction (2), the hydrogen storage capacity for n =6 is 5.46% as compared with 6.56% for AE. Thus, the unknown generation of GA and hydrogen from AE is an important challenge, as is the unknown hydrogenation of GA; hydrogenation of diketopiperazines was never reported, under any conditions, be it under homogeneous or heterogeneous catalysis or any pressure. Initially, 10 mmol of AE was heated at 135 °C under argon for 12 h in the absence of solvent with 0.05 mol% of 1 and 0.06 mol% of KO t Bu (for the in situ generation of the active catalyst 2 ), resulting in no product formation ( Table 1 , entry 1). However, using 10 mmol of AE and 0.5 mol% of catalyst 1 with no solvent resulted in 48% conversion to mostly linear peptides, and 25% yield of H 2 (entry 2). Adding 0.5 ml dioxane as a solvent to 1 mmol of AE using catalyst loading of 0.5 mol% resulted in 57% conversion of AE to linear peptides as the major products, as observed by nuclear magnetic resonance (NMR) spectroscopy and mass spectrometry (entry 3). Significantly, using 2 ml dioxane as solvent and 0.5 mol% of catalyst 1 , 68% conversion was observed, forming GA in 31% yield, the rest being linear peptides (entry 4). Increasing the volume of dioxane led to improvement in both the yield of GA and the amount of linear products (entries 4–6). However, using >4 ml dioxane was not beneficial (entries 10 and 11). Use of the bipyridine-based pincer complexes 3 and 4 resulted in much lower conversion of AE (entries 7 and 8). Table 1 Selected results of optimization studies for dehydrogenation of 2-aminoethanol. Full size table Next, we used the PNN-H complex 5 (ref. 28 ), bearing an N(H)( t Bu) amine group instead of the NEt 2 group in 1 . It was hoped that the presence of an NH group might allow for metal–ligand cooperation via the well-known Ru-amino/Ru-amido sequence [29] in addition to metal–ligand cooperation via aromatization–dearomatization of the pincer ligand [22] , [23] , [24] , [25] , [26] . However, use of 1.2 equiv. of base (relative to 5) resulted in similar conversion of AE and lower yield of GA (entry 9). Importantly, increasing the base loading resulted in much higher catalytic efficiency. Thus, using 0.5 mol% of 5 and 1.2 mol% of KO t Bu (2.4 equiv. relative to 5 ) resulted in 85% conversion of AE and 60% yield of GA (entry 14) with formation of 37 ml of H 2 , corresponding to 77% yield of hydrogen based on the reaction of Fig. 1c . Two equivalents of base relative to 5 likely lead to deprotonation of both the amine group and the benzylic arm ( Supplementary Note 1 ) [28] . Higher base loadings (entries 15 and 16) and lower temperatures (entries 17 and 18) led to lower GA yields. Increased base loading also led to lower yields of GA when using catalyst 1 ( c.f. entries 6 and 19). The dehydrogenation reaction was also tried in a large scale of 20 mmol under the conditions of entry 14, of which give similar results, namely 89% conversion of AE, 55% yield of GA and 74% of H 2 (710 ml; entry 20). Using mixtures of dioxane with polar or nonpolar solvents, including diglyme, dimethylformamide, valeronitrile, dimethylacetamide, N -methylmorpholine and toluene resulted in lower catalytic efficiencies ( Supplementary Table 3 ). 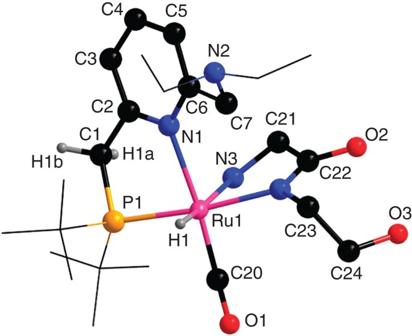Figure 3: X-ray structure of complex 8. Hydrogen atoms (except hydride and the hydrogen atoms on C1) are omitted for clarity.tBu and Et groups are presented as wireframe (seeSupplementary Fig. 2for a different perspective). Selected bond lengths (Å) and angles (°): Ru(1)-C(20) 1.809(3), Ru(1)-N(4) 2.147(2), Ru(1)-N(3) 2.232(3), Ru(1)-N(1) 2.248(3), Ru(1)-P(1) 2.2733(8), Ru(1)-H(1) 1.7275, C(1)-C(2) 1.506(4), C(6)-C(7) 1.510(4), C(22)-O(2) 1.273(4), C(24)-O(3) 1.414(4); C(20)-Ru(1)-N(4) 90.33(11), C(20)-Ru(1)-N(3) 100.93(13), N(4)-Ru(1)-N(3) 75.75(9), C(20)-Ru(1)-N(1) 174.84(12), N(4)-Ru(1)-N(1) 94.33(9), N(3)-Ru(1)-N(1) 82.39(10), N(4)-Ru(1)-P(1) 172.46(7), N(3)-Ru(1)-P(1) 98.22(7), N(1)-Ru(1)-P(1) 80.23(7). Using no solvent or a very small amount of solvent also resulted in lower efficiency of the dehydrogenative coupling reaction, although substantial dehydrogenation was still observed ( Supplementary Table 4 and Supplementary Note 2 ). 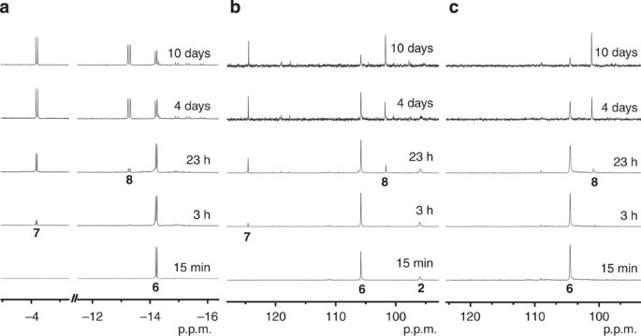Figure 4: Reaction of complex 2 with AE at r.t. in C6D6. (a)1H NMR spectra using 1.5 equiv. of AE, (b)31P{1H} NMR spectra using 1.5 equiv. of AE and (c)31P{1H} NMR spectra using 10 equiv. of AE. For example, heating a mixture of only 0.1 ml dimethyl sulfoxide solvent and 10 mmol AE (0.611 ml) with 0.5 mol% catalyst 1 and 0.6 mol% KO t Bu at 170 °C for 12 h resulted in 71% conversion of AE, mostly to linear oligopeptides, and 39% yield of H 2 (55% relative to converted AE based on the reaction in Fig. 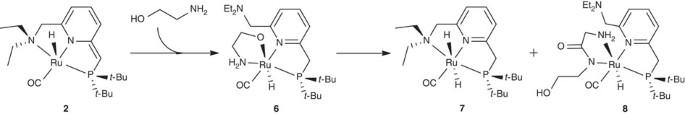1c and Supplementary Table 4 , entry 8). Hydrogenation experiments Catalysts 1 and 5 were tested for the hydrogenation of GA, which is unprecedented for any diketopiperazine. Figure 2: Observed path from complex 2 to complexes 6, 7 and 8.  No product was obtained under 10 bar of H 2 in tetrahydrofuran (THF) using 1 mol% catalyst at 110 °C ( Table 2 , entries 1 and 2). Applying 50 bar of H 2 , 2 mol% of catalyst 1 and 2.4 mol% KO t Bu in dioxane at 110 °C resulted in quantitative yield of the linear amide 2-amino- N -(2-hydroxyethyl)acetamide (AA; entry 3; ref. 30 ). Using more base improved the reaction significantly; 61% yield of AE and 34% yield of AA were produced using 4.8 mol% KO t Bu and 2 mol% catalyst 1 (entry 4). Importantly, complex 5 was catalytically much more active than 1 and nearly 100% yield of the desired AE was obtained, even when only 0.5 mol% 5 and less solvent were used (entries 5 and 6). However, lower H 2 pressure (20 bar) was ineffective (entry 7). The mixed products of GA and linear peptides produced by the dehydrogenative reaction (under conditions of Table 1 , entry 14) were also hydrogenated by catalyst 5 , leading to 85 wt% yield of AE under 50 bar of H 2 (entry 8). Thus, formation of linear peptides does not pose a significant problem regarding regeneration of AE. Higher pressure of H 2 was not beneficial (entry 9). A larger amount of GA (5 mmol) was also hydrogenated successfully under 70 bar of H 2 in a shorter time (12 h) and less solvent (5 ml dioxane for 5 mmol GA), resulting in full conversion of GA, 96% yield of AE and 4% yield of AA (entry 10). Table 2 Selected optimization results for the hydrogenation of glycine anhydride. Full size table Repetitive reversal reactions Repetitive cycles of the dehydrogenation–hydrogenation reactions were also tried without adding new catalyst ( Table 3 , see Supplementary Methods for procedure details). 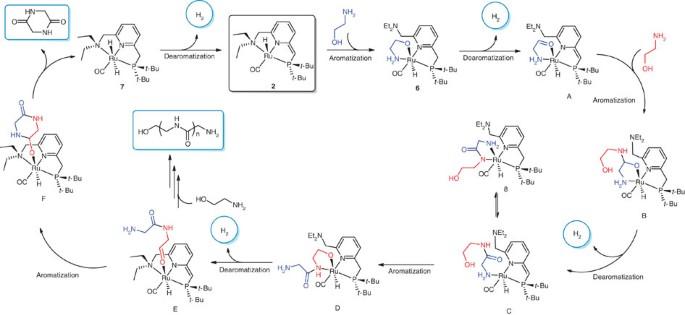Figure 5: Proposed mechanism for dehydrogenative coupling of AE catalysed by complex 2.  The cycles began with dehydrogenation, using 1 mol% catalyst 5 , 2.4 mol% KO t Bu, 1 mmol 2-AE and 4.5 ml dioxane (for an example of applying 0.5 mol% catalyst, see Supplementary Methods and Supplementary Table 5 for details). A catalytic amount of KO t Bu (2.4 equiv. relative to complex 5 ) was added every time after the former reaction, to protect the catalyst from trace amount of water, which may be taken into the system during the course of transfer (catalysed by PNN ruthenium pincer complexes, water and alcohol can produce a carboxylic acid [31] , which can poison the catalyst in the absence of base). After the first dehydrogenation reaction, of which 86% conversion of AE was achieved, the crude reaction mixture was transferred to a 20-ml Parr apparatus under N 2 atmosphere. The Parr apparatus was then filled with H 2 and the hydrogenation reaction was performed. Without isolation, the catalytic activity of the system was higher as compared with Table 2 , entry 9 and 97% of AE (based on the amount of AE used in the first dehydrogenation reaction) was observed. Following this, the second dehydrogenation step resulted in 79% conversion of AE, while the second hydrogenation step provided 90% of AE. The results of the third cycle were also good, even after using the catalyst for six times, 81% of AE was still observed at the end of the third hydrogenation step. Table 3 Repetitive cycles of the dehydrogenation–hydrogenation reactions. Full size table Mechanistic experiments To gain mechanistic understanding, the reaction of the dearomatized complex 2 with AE was studied by NMR spectroscopy ( Supplementary Note 3 ). Addition of 1.5 equiv. of AE to a C 6 D 6 solution of 2 at room temperature (r.t.) rapidly afforded nearly quantitatively the aromatic alkoxo species 6 ( Fig. 2 ), which exhibits a hydride signal (d, −14.22 p.p.m., J PH =18.9 Hz) in 1 H NMR and a singlet at ∼ 106 p.p.m. in 31 P{ 1 H} NMR. The signals of the two NH 2 protons appear at very different chemical shifts in 1 H NMR (4.58 and 2.83 ppm) as previously observed for related complexes [29] , while the two methyl groups of NEt 2 exhibit a single triplet (6 H, 0.86 p.p.m., J HH =7.1 Hz); both these observations indicate coordination of the NH 2 group of AE and decoordination of the NEt 2 ‘arm’. Complex 6 is stable below −30 °C and slowly decomposes at r.t. to the known trans -dihydride complex 7 (ref. 23 ) and to a new species ( 8 ). Complex 7 is likely formed by hydride elimination from complex 6 ( Fig. 2 ). Complex 8 exhibits a singlet at ∼ 102 p.p.m. in 31 P{ 1 H} NMR and a hydride signal at −13.16 p.p.m. (d, J PH =23.2 Hz) in 1 H NMR. Crystals of 8 suitable for X-ray analysis were obtained by pentane diffusion into a concentrated benzene solution of 6 . Complex 8 has a distorted octahedral geometry around the Ru(II) centre ( Fig. 3 ), with the phosphorus atom coordinated trans to the nitrogen atom of the amide group and the hydride located trans to the NH 2 group. The two nitrogen atoms of the N–C–C–N backbone form a five-membered chelate. The C–C bond lengths (C(2)–C(3) 1.388(5), C(3)–C(4) 1.391(5) Å) indicate that complex 8 is aromatized ( Fig. 3 ), consistent with the NMR data. The amide backbone is formed by dehydrogenative coupling of two molecules of AE, illustrating highly selective amide rather than ester formation. Figure 2: Observed path from complex 2 to complexes 6, 7 and 8. Full size image Figure 3: X-ray structure of complex 8. Hydrogen atoms (except hydride and the hydrogen atoms on C1) are omitted for clarity. t Bu and Et groups are presented as wireframe (see Supplementary Fig. 2 for a different perspective). Selected bond lengths (Å) and angles (°): Ru(1)-C(20) 1.809(3), Ru(1)-N(4) 2.147(2), Ru(1)-N(3) 2.232(3), Ru(1)-N(1) 2.248(3), Ru(1)-P(1) 2.2733(8), Ru(1)-H(1) 1.7275, C(1)-C(2) 1.506(4), C(6)-C(7) 1.510(4), C(22)-O(2) 1.273(4), C(24)-O(3) 1.414(4); C(20)-Ru(1)-N(4) 90.33(11), C(20)-Ru(1)-N(3) 100.93(13), N(4)-Ru(1)-N(3) 75.75(9), C(20)-Ru(1)-N(1) 174.84(12), N(4)-Ru(1)-N(1) 94.33(9), N(3)-Ru(1)-N(1) 82.39(10), N(4)-Ru(1)-P(1) 172.46(7), N(3)-Ru(1)-P(1) 98.22(7), N(1)-Ru(1)-P(1) 80.23(7). Full size image An NMR study of the reaction of catalyst 2 with 10 equiv. of AE at r.t. ( Fig. 4c ) showed formation of complexes 6 and 8 as the major species, and after 10 days 8 became the major product. Compared with reaction of complex 2 with 1.5 equiv. of AE ( Fig. 4b ), complex 7 was nearly fully consumed when 10 equiv. of AE were used. Complex 8 was also independently prepared by reaction of 2 with AA ( Supplementary Methods ). In addition, complex 8 was catalytically active for the dehydrogenation of AE under the conditions in which complex 1 was used, resulting in 81% conversion of AE to GA (33% yield) and linear peptides (see Supplementary Methods for details). Figure 4: Reaction of complex 2 with AE at r.t. in C 6 D 6 . ( a ) 1 H NMR spectra using 1.5 equiv. of AE, ( b ) 31 P{ 1 H} NMR spectra using 1.5 equiv. of AE and ( c ) 31 P{ 1 H} NMR spectra using 10 equiv. of AE. Full size image On the basis of the NMR studies, the isolation of complex 8 , and the known chemistry of pyridine-based pincer ruthenium complexes [22] , [23] , [24] , [25] , [26] , the mechanism shown in Fig. 5 is proposed. Reaction of the dearomatized complex 2 with AE leads to the aromatic alkoxy complex 6 . Following dehydrogenation by metal–ligand cooperation, the 2-amino aldehyde intermediate A is formed and then attacked by another molecule of AE, providing the aromatic hemi-aminoxy intermediate B . Subsequent hydride elimination and H 2 generation affords the dearomatized AA-intermediate C . Isomerization of C and activation of the O–H bond produces the aromatic species D , followed by hydride elimination to generate an aldehyde group and release a third molecule of H 2 to afford intermediate E . Intramolecular reaction between the amino and aldehyde groups in complex E produces GA via intermediate F , while an intermolecular reaction with AE results in a linear oligopeptide. During formation of D from intermediate C , isomerization followed by amide N–H activation produces complex 8 . Figure 5: Proposed mechanism for dehydrogenative coupling of AE catalysed by complex 2. Full size image In summary, we have developed a fundamentally new, reversible system that can load and unload H 2 with a potentially high hydrogen storage capacity. It is based on a unique acceptorless dehydrogenative coupling process involving cheap and abundant AE, and hydrogenation of the product cyclic dipeptide GA, which takes place with the same catalyst system. Insight into the mechanism is provided, including isolated intermediates. Although there are limitations at this early stage, we believe that this fundamental system provides a sound basis for the development, upon further improvements, such as solvent elimination, of an attractive LOHC system based on inexpensive, abundant and safe AE carrier. The success of this system highlights the possibilities of applying fundamentally new chemical reactions, such as reversible acceptorless peptide bond formation, as a basis for novel LOHCs. See Supplementary Methods and Supplementary Fig. 3 for general procedures and further details. Accession codes : The X-ray crystallographic coordinate for the structure (complex 8 ) reported in this Article has been deposited at the Cambridge Crystallographic Data Centre (CCDC), under deposition number CCDC 1017722. The data can be obtained free of charge from The Cambridge Crystallographic Data Centre via www.ccdc.cam.ac.uk/data_request/cif . How to cite this article: Hu, P. et al. A novel liquid organic hydrogen carrier system based on catalytic peptide formation and hydrogenation. Nat. Commun. 6:6859 doi: 10.1038/ncomms7859 (2015).